Coherent anti-Stokes Raman scattering with single-molecule sensitivity using a plasmonic Fano resonance Plasmonic nanostructures are of particular interest as substrates for the spectroscopic detection and identification of individual molecules. Single-molecule sensitivity Raman detection has been achieved by combining resonant molecular excitation with large electromagnetic field enhancements experienced by a molecule associated with an interparticle junction. Detection of molecules with extremely small Raman cross-sections (~10 −30 cm 2 sr −1 ), however, has remained elusive. Here we show that coherent anti-Stokes Raman spectroscopy (CARS), a nonlinear spectroscopy of great utility and potential for molecular sensing, can be used to obtain single-molecule detection sensitivity, by exploiting the unique light harvesting properties of plasmonic Fano resonances. The CARS signal is enhanced by ~11 orders of magnitude relative to spontaneous Raman scattering, enabling the detection of single molecules, which is verified using a statistically rigorous bi-analyte method. This approach combines unprecedented single-molecule spectral sensitivity with plasmonic substrates that can be fabricated using top-down lithographic strategies. Raman spectroscopy measures the vibrational modes of a molecule, providing information about its molecular structure, conformation and temperature. Surface-enhanced Raman scattering (SERS) [1] , [2] , [3] has advanced to the detection limit of individual resonant molecules when the molecule is closely associated with the nanoscale junction between chemically fabricated nanoparticles [4] , [5] , [6] , [7] , [8] , [9] , [10] , [11] , [12] . Here two enhancement mechanisms are at play: the enhanced Raman cross-section of a molecule when the excitation laser is resonant with an electronic excitation of the molecule; and the extremely large local electromagnetic (EM) field enhancement generated by optically exciting the collective plasmon mode of the two closely adjacent nanoparticles. Due to the magnitude of the EM enhancement achievable in nanoparticle junctions, it appears doubtful whether this same approach could be used to generally detect random ‘unknown’ molecules at the single-molecule level. One could, however, improve molecular detection sensitivity further by combining plasmonic (SERS) enhancements with coherence. Coherent anti-Stokes Raman scattering (CARS) [13] , [14] , [15] , [16] , [17] is a third-order nonlinear optical process (a specific type of four-wave mixing (FWM) spectroscopy) that employs molecular coherence. In CARS, the pump ( ω P ) and Stokes ( ω S ) fields interact coherently through the third-order polarizability of the dipole-forbidden vibronic modes of a molecule, generating an anti-Stokes signal ω AS =2 ω P − ω S with the intensity dependence of a third-order nonlinear optical process: When the frequency difference ω P − ω S coincides with a Raman (dipole-forbidden vibrational) band of the molecule, the CARS signal is resonantly enhanced as a scattering peak. This two-beam, coherent process is usually orders of magnitude stronger than spontaneous Raman scattering [18] . Coherent and spontaneous Raman scattering processes are diagrammed in Fig. 1a . 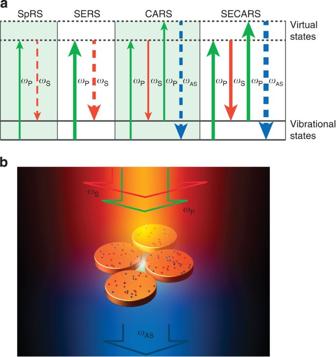Figure 1: Different types of Raman processes and the SECARS configuration. (a) Energy level diagram shows four types of Raman processes of a molecule. The arrow thickness indicates the transition strength. (b) SECARS configuration of two diluted molecules on a nanoquadrumer. A single-wavelength pump laser (ωP) and a supercontinuum Stokes laser (ωS) generate an enhanced anti-Stokes scattering (ωS) of a molecule in the quadrumer central gap. Figure 1: Different types of Raman processes and the SECARS configuration. ( a ) Energy level diagram shows four types of Raman processes of a molecule. The arrow thickness indicates the transition strength. ( b ) SECARS configuration of two diluted molecules on a nanoquadrumer. A single-wavelength pump laser ( ω P ) and a supercontinuum Stokes laser ( ω S ) generate an enhanced anti-Stokes scattering ( ω S ) of a molecule in the quadrumer central gap. Full size image The sensitivity of CARS can be increased even further by designing an appropriately resonant plasmonic substrate. If the input ( ω P , ω S ) or output ( ω AS ) frequencies in CARS are in resonance with the collective modes of the plasmonic nanostructure, the surface-enhanced CARS (SECARS) [18] , [19] , [20] , [21] signal from molecules adsorbed onto the nanostructure will be further enhanced by the local fields of the excited plasmon modes. The EM enhancement factor in SECARS is given by the product of the enhanced local EM fields at the characteristic frequencies of the spectroscopy: an appropriate plasmonic substrate for CARS would provide EM enhancements at these three characteristic frequencies. In this Article, we show that plasmonic nanostructures supporting Fano resonances can be designed to enhance the CARS with single-molecule sensitivity. Plasmonic Fano resonances by their nature as coupled subradiant and superradiant modes can provide much larger field enhancements than bright modes [22] , [23] , [24] , [25] , [26] . The substrate we use is a quadrumer, that is, four coupled nanodisks ( Fig. 1b ) that possess a strong Fano resonance [27] . The local fields give rise to a highly localized SECARS enhancement in a single junction at the center of the quadrumer structure, a field distribution particularly well suited for achieving single-molecule detection sensitivity. We verify SECARS of single molecules with Raman cross-sections as low as 10 −30 cm 2 sr −1 , using a bi-analyte method. SECARS substrates and experimental setup The plasmonic quadrumer [27] ( Fig. 2a , inset) is composed of four Au disks of diameter 158.9±2.2 nm and height 51.1±2.5 nm with an interparticle spacing of 15.4±1.1 nm, evaporated onto a fused silica substrate (see Methods). The optical spectrum of a plasmonic quadrumer cluster clearly shows a strong Fano resonance due to its coupled subradiant and superradiant plasmon modes ( Fig. 2a ). Its linear (Rayleigh) scattering spectrum ( Fig. 2a ) reveals a narrow minimum centered at ~772 nm on top of a far broader resonance, which red-shifts to ~800 nm after functionalization of a monolayer of para -mercaptoaniline ( p -MA) molecules. To exploit these spectral properties for SECARS, it is most advantageous to minimize losses at the pump wavelength while maximizing far-field coupling for the wavelength range of the anti-Stokes emission. The reduction of scattered light at frequencies corresponding to the Fano dip maximizes energy coupling into the structure at those frequencies ( Fig. 2a , wavelength marked in green). For the anti-Stokes output light, the superradiant shoulder of the optical spectrum acts as an antenna, maximizing the propagation of the anti-Stokes light to the far field ( Fig. 2a , blue wavelength band). 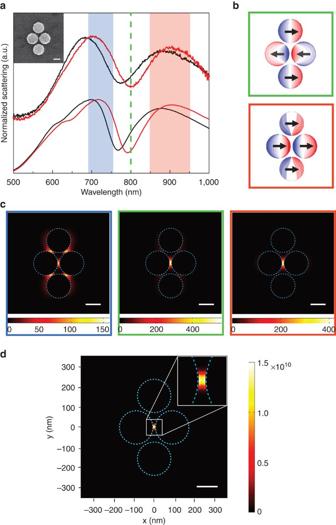Figure 2: Experimental and FDTD simulated properties of the quadrumer withp-MA molecule monolayer coating. (a) Experimental (top) and calculated (bottom) linear scattering spectra of a single quadrumer before (black) and after (red) thep-MA absorption, obtained with horizontal polarization. The calculated spectra for both cases are consistent with their corresponding experimental results. Green dashed line: the pump beam (800 nm); red zone: the Stokes scattering region (848–952 nm); blue zone: the anti-Stokes scattering region (756–690 nm). The Stokes and anti-Stokes regions correspond to Raman shifts of 700–2,000 cm−1. The inset shows an s.e.m. image of a gold quadrumer. (b) Charge densities on the top surface of the quadrumer excited at 800 nm pump (top) and 900 nm Stokes (bottom), corresponding to the subradiant and superradiant modes, respectively. (c) Field enhancement intensity (g2) distribution at the anti-Stokes (left), pump (middle) and Stokes (right) frequencies for thep-MA 1,070 cm−1mode evaluated at mid-height of the quadrumer. (d) SECARS enhancement (GSECARS=gP4gS2gAS2) map for the mode inc. The maximum enhancement factor is ~1.5 × 1010in the central gap, and significantly lower (~2.5 × 106) in the four peripheral gaps. Scale bar, 100 nm. FDTD, finite-difference-time-domain. Figure 2: Experimental and FDTD simulated properties of the quadrumer with p -MA molecule monolayer coating. ( a ) Experimental (top) and calculated (bottom) linear scattering spectra of a single quadrumer before (black) and after (red) the p -MA absorption, obtained with horizontal polarization. The calculated spectra for both cases are consistent with their corresponding experimental results. Green dashed line: the pump beam (800 nm); red zone: the Stokes scattering region (848–952 nm); blue zone: the anti-Stokes scattering region (756–690 nm). The Stokes and anti-Stokes regions correspond to Raman shifts of 700–2,000 cm −1 . The inset shows an s.e.m. image of a gold quadrumer. ( b ) Charge densities on the top surface of the quadrumer excited at 800 nm pump (top) and 900 nm Stokes (bottom), corresponding to the subradiant and superradiant modes, respectively. ( c ) Field enhancement intensity ( g 2 ) distribution at the anti-Stokes (left), pump (middle) and Stokes (right) frequencies for the p -MA 1,070 cm −1 mode evaluated at mid-height of the quadrumer. ( d ) SECARS enhancement ( G SECARS = g P 4 g S 2 g AS 2 ) map for the mode in c . The maximum enhancement factor is ~1.5 × 10 10 in the central gap, and significantly lower (~2.5 × 10 6 ) in the four peripheral gaps. Scale bar, 100 nm. FDTD, finite-difference-time-domain. Full size image The nature and origin of the Fano resonance can be better understood by examining the surface charge densities at different wavelengths associated with this resonance ( Fig. 2b ). The Fano resonance is a result of interference between a subradiant mode and a superradiant mode. For the resonant frequency of the Fano dip, dipoles of the left and right nanodisks oscillate out of phase with the top and bottom disks in this symmetry-breaking quadrumer ( Fig. 2b , green), indicating a small net dipole moment and subradiant behaviour. For the broad plasmon peak, the dipoles of all four disks oscillate in phase, indicating superradiant behaviour ( Fig. 2b , red). The pronounced Fano dip in the otherwise superradiant scattering continuum indicates resonant energy storage at the frequencies corresponding to this feature [27] . By optimizing the nanodisk diameters and gap sizes, we can tune the plasmonic quadrumer geometry so that its Fano resonance corresponds to the frequency of the pump laser; then the superradiant shoulders to the red and blue of the Fano minimum correspond to the Stokes and anti-Stokes scanning regions of the SECARS spectrum, respectively. These simultaneous resonances in the same spatial location result in a ‘mixed frequency coherent mode’ as previously described on more complex plasmonic clusters [22] . The field intensity distributions for the plasmonic quadrumer at the pump, Stokes and anti-Stokes frequencies, for the 1,070 cm −1 Raman mode of the adsorbate molecule p -MA, are shown in Fig. 2c . The strong spatial localization at all three frequencies leads to a tightly confined ‘SECARS hot spot’ in the center of the cluster with an ~250 nm 2 size (only ~0.31% of the surface area of a quadrumer) ( Fig. 2d ). With horizontally polarized excitation, the four peripheral gaps have a SECARS enhancement ~6,000 times weaker than the central gap, thus a large CARS polarization could be effectively induced only by the molecules located in the region of this central gap. In this region, we calculated that the SECARS over CARS enhancement is ~1.5 × 10 10 for this mode, and is 0.7–2.3 × 10 10 for Raman modes spanning the range of 700–2,000 cm −1 ( Supplementary Fig. 1 ). In comparison, SERS on this same structure and pump laser frequency was calculated to enhance only ~2.5 × 10 5 over spontaneous Raman scattering. It is also useful to compare the SECARS enhancement (over CARS) for this Fano-resonant cluster with other plasmonic but non-Fano clusters: SECARS by a broadly resonant (non-Fano) plasmonic quadrumer is enhanced by ~7.5 × 10 8 over unenhanced CARS ( Supplementary Fig. 2 ); SECARS by a nanovoid gold surface [18] is enhanced ~10 5 over CARS when all frequencies coincide with its plasmon resonances. Taking into consideration that CARS is usually orders of magnitude stronger than spontaneous Raman [18] , SECARS due to this Fano-resonant quadrumer should be anticipated to be enhanced more than 10 orders of magnitude over the spontaneous Raman process. In the SECARS experiments, one laser beam from a single 76 MHz pulsed Ti:sapphire oscillator was split into two beams, consisting of a pump beam and a continuum Stokes beam, the latter generated by propagating a fraction of the beam through a nonlinear photonic crystal fibre. These two horizontally polarized, collinear and coherent pulse trains were focused onto the sample, which was mounted on a microscope with a high-precision positioning stage to place the desired quadrumer at the laser focus (Methods and Supplementary Fig. 3 ). The focused laser spot was ~1 μm in diameter, where both incident beams behave like normal-incident plane waves on the quadrumer surface [22] . The CARS emission was collected by an objective in transmission and analysed by a spectrometer. When the CARS polarizations are generated in a volume much smaller than its propagation wavelength, and/or in the focused laser fields, the phase matching requirements for nonlinear optics can be fulfilled automatically (|Δ k × z <<π| when z << λ ) [16] , [28] . Ensemble-molecule detection We first performed SECARS with this quadrumer structure on ensemble molecules (see Methods). The input ( Fig. 3a ) consisted of a pump beam centered at ω P =800 nm, and a Stokes continuum ω S =830–1,050 nm spanning several hundred nanometers to the long wavelength side of the pump wavelength. Several types of molecules nonresonant at these laser excitation wavelengths have been investigated ( Supplementary Fig. 4 ). The resulting spectrum ( Fig. 3b ) from p -MA molecules (~10 3 molecules bound to the Au surfaces of the probe region of the quadrumer structure) consists of three sharp anti-Stokes features on top of a broadband background. The background has two main contributions: a dominant two-photon luminescence signal [29] , [30] , as well as a much weaker FWM signal [22] , both due to the Au nanostructure ( Supplementary Fig. 5 and Supplementary Note 1 ). These background signals were measured before the SECARS experiments on a pristine quadrumer sample. The applied laser power was too low to affect the stability of the molecule, thus the output spectra were stable during the ~10-min acquisition time. Interestingly, the CARS spectrum of p -MA showed quadrumer-to-quadrumer variations, characteristic of a depolarization behaviour with random fluctuations, likely due to variable orientations of molecules within the gap [31] , [32] . 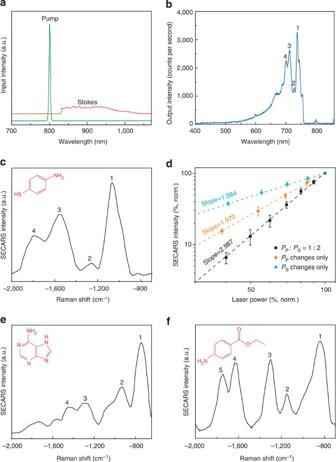Figure 3: SECARS experiments of ensemble molecules on the quadrumer. (a) Input spectra of the pump (green) and Stokes (red) beams. (b) Example output signal ofp-MA obtained withPP=33 μW andPS=67 μW. The numbers of photons were recorded with pixel size ~0.4 nm. (c) Reconstructed SECARS spectrum versus Raman shift ofp-MA shows two prominent peaks at −1,070 cm−1(1) and −1,580 cm−1(3), a weak charge-transfer mode at approximately −1,290 cm−1(2) and an overtone of ring mode at approximately −1,800 cm−1(4), all corresponding to peaks with same numbers inb. (d) Normalized (norm.) peak power at −1,070 cm−1versus normalized total inputPtot(black squares,Ptot=40–100 μW withP1:P2=1:2),PPchange only (orange circles,PP=13–33 μW withPS=67 μW) andPSchange only (cyan triangles,PS=27–67 μW withPP=33 μW) on a log-log scale.PSrepresents the overall power of continuum wavelengths. Dashed lines are linear fitting functions. Error bars represent standard deviations ofp-MA CARS signals on five individual quadrumers. (e) SECARS spectrum of adenine shows four expected peaks at −740 cm−1(1), −950 cm−1(2), −1,270 cm−1(3) and −1,450 m−1(4). (f) SECARS spectrum of benzocaine shows five expected peaks at −850 cm−1(1), −1,160 cm−1(2), −1,290 cm−1(3), −1,610 cm−1(4) and −1,700 cm−1(5). Figure 3: SECARS experiments of ensemble molecules on the quadrumer. ( a ) Input spectra of the pump (green) and Stokes (red) beams. ( b ) Example output signal of p -MA obtained with P P =33 μW and P S =67 μW. The numbers of photons were recorded with pixel size ~0.4 nm. ( c ) Reconstructed SECARS spectrum versus Raman shift of p -MA shows two prominent peaks at −1,070 cm −1 (1) and −1,580 cm −1 (3), a weak charge-transfer mode at approximately −1,290 cm −1 (2) and an overtone of ring mode at approximately −1,800 cm −1 (4), all corresponding to peaks with same numbers in b . ( d ) Normalized (norm.) peak power at −1,070 cm −1 versus normalized total input P tot (black squares, P tot =40–100 μW with P 1 : P 2 =1:2), P P change only (orange circles, P P =13–33 μW with P S =67 μW) and P S change only (cyan triangles, P S =27–67 μW with P P =33 μW) on a log-log scale. P S represents the overall power of continuum wavelengths. Dashed lines are linear fitting functions. Error bars represent standard deviations of p -MA CARS signals on five individual quadrumers. ( e ) SECARS spectrum of adenine shows four expected peaks at −740 cm −1 (1), −950 cm −1 (2), −1,270 cm −1 (3) and −1,450 m −1 (4). ( f ) SECARS spectrum of benzocaine shows five expected peaks at −850 cm −1 (1), −1,160 cm −1 (2), −1,290 cm −1 (3), −1,610 cm −1 (4) and −1,700 cm −1 (5). Full size image Figure 3c shows the reconstructed SECARS spectrum of p -MA, obtained by averaging three output spectra at different pump-Stokes delays ( Supplementary Fig. 6 and Supplementary Note 2 ), correcting (subtracting) for background noise ( Supplementary Fig. 5a ), and calibrated (divided) by the quadrumer SECARS enhancement [33] ( Supplementary Fig. 1b ) and instrument efficiency spectrum at each wavelength. The obtained spectra in wavelengths ( λ ) were then converted into wavenumbers ( k ) by the following equation: Δ k =10 7 × (1/800–1/ λ ). The broad Raman peaks (~100 cm −1 ) are mostly due to the spectral bandwidth of the pump (~5 nm). Two prominent p -MA modes due to the EM field enhancement [23] , a peak at approximately −1,800 cm −1 due to the overtone of the ring mode [34] , and a weak mode at ~1,290 cm −1 possibly due to the combined contribution of CT (charge-transfer between Au surface and adsorbed molecules) and EM mechanisms can be observed. See Supplementary Fig. 7 for the control experiments of normal Raman and SERS, Supplementary Tables 1–3 for complete Raman-band assignments and Supplementary Note 3 for the explanation of the CT contribution. The intensity of the −1,070 cm −1 p -MA mode ( Fig. 3d ) was observed to depend cubically on the total input power P tot , quadratically on the pump power P P , and linearly with Stokes power P S . These results follow the third-order nonlinearity scaling of equation (1), further confirming the CARS origin of the spectrum, and demonstrate that the intensities in our experiment have not reached the coherent-Raman saturation threshold [35] . Using this approach we were able to obtain SECARS spectra from a variety of other small molecules. The SECARS spectrum of adenine, one of the constituent bases of DNA and RNA, is dominated by the −740 cm −1 ring-breathing mode [36] ( Fig. 3e ). Benzocaine, another polyheterocyclic aromatic molecule, has a SECARS spectrum ( Fig. 3f ) characterized by five primary modes [37] . The clearly resolvable features of these SECARS spectra indicate the potential for vibrational spectroscopy of these and similar molecular species in ultrasmall quantities. Single-molecule detection We then examined whether SECARS obtained using this approach could achieve single-molecule sensitivity for small molecules, which would require [38] an enhancement factor of ~10 10 –10 11 . A polarization-sensitive CARS geometry [39] (with a polarization analyser oriented to transmit y -polarized light placed before the detector) was used to suppress ~99% of the essentially x -polarized [22] background FWM signal, with the quadrumer dimensions slightly modified to reduce the unpolarized background two-photon luminescence ( Supplementary Fig. 8 and Supplementary Note 4 ). We used the bi-analyte method [7] , [10] , where p -MA and adenine (both Raman cross-sections ~10 −30 cm 2 sr −1 in air for NIR excitation [38] , [40] ) have clearly distinguishable Raman spectra allowing for the unequivocal identification of each molecule. A mixed solution of equal concentrations (100 nM) of the two molecules was drop-casted onto multiple (49) quadrumers for SECARS. This concentration was chosen to ensure that ~1.5 molecules fall into each probe region (250 nm 2 area; 6,250 nm 3 volume) onto the substrate [7] , [10] , based on our estimation (see Methods). Each molecule type should have similar probability of deposition by the drop-casting method at this sufficiently low coverage, as two molecules will not compete for binding on the Au surface due to their very large separation ( Supplementary Fig. 9 and Supplementary Note 5 ). Typical SECARS spectra from three of the measured quadrumers are shown in Fig. 4a (see Supplementary Fig. 10 and Supplementary Note 6 for raw spectra). Two of the spectra shown here correspond extremely closely to the p -MA and adenine SECARS spectra obtained using higher concentrations of each of those respective adsorbate molecules. The ‘mixed’ spectrum clearly has spectral features that correspond to the spectra of both molecules. At these concentrations, we observed good Raman-band reproducibility among quadrumers with fluctuations in intensities, frequencies and spectral features ( Supplementary Fig. 11 ), most likely due to different molecular orientations with respect to the analyser and laser polarization, a characteristic that we believe to be a signature of single or a few molecules. In contrast to more concentrated solutions of the two analyte molecules which should always yield a mixed spectrum, we observed, for a series of 49 quadrumers, that the SECARS spectra were dominated by either one analyte or the other, or no molecules detected at all ( Fig. 4b ). At low concentration, the number of molecules in each probe region should follow a Poisson distribution [7] , [10] with an expected value μ . We obtained μ =0.89±0.24 by fitting the measured data ( Supplementary Note 7 ), close to our estimated value of 1.5. Based on the measured signal intensities, our SECARS is ~10 11 times stronger than the spontaneous Raman scattering signal from these molecules ( Supplementary Note 8 ). From our experimental measurements, the SECARS probe region is estimated to be roughly ~167 nm 2 in area (4,175 nm 3 in volume), only 0.19% of the entire quadrumer surface area (volume), close to the simulation result of 250 nm 2 area (6,250 nm 3 volume). These observations all provide clear evidence that SECARS obtained in this manner provides single-molecule sensitivity. 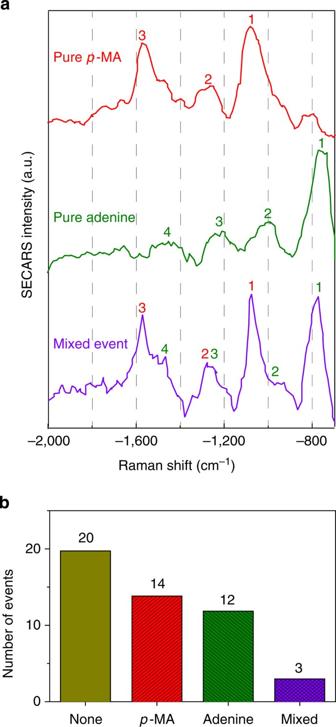Figure 4: Single-molecule SECARS detection of bianalytes. (a) Three representative SECARS spectra showing a purep-MA event (top), a pure adenine event (middle) and a mixed event (bottom). (b) Histogram of occurrences of none, purep-MA, pure adenine and mixed molecules from one sampled array of 49 quadrumers. Figure 4: Single-molecule SECARS detection of bianalytes. ( a ) Three representative SECARS spectra showing a pure p -MA event (top), a pure adenine event (middle) and a mixed event (bottom). ( b ) Histogram of occurrences of none, pure p -MA, pure adenine and mixed molecules from one sampled array of 49 quadrumers. Full size image In conclusion, we have demonstrated SECARS utilizing a Fano-resonant plasmonic quadrumer substrate, which provides an ~10 11 enhancement over spontaneous Raman scattering, and is capable of single-molecule sensitivity with Raman cross-sections σ Raman as low as ~10 −30 cm 2 sr −1 . These values are among the smallest values for molecules (except perhaps for N 2 and alkane molecules, which have σ Raman ~10 −31 and 10 −32 cm 2 sr −1 , respectively, at NIR excitations [38] , [41] ). Obtaining single-molecule spectra using a substrate that can be fabricated with standard lithographic methods can, in principle, ultimately open the door to the identification of unknown molecules at the ultimate limits of chemical sensitivity. Such ultimate detection thresholds could have tremendous applicability in fields as diverse as medical diagnostics, forensics, and homeland security. SECARS substrates The quadrumers were fabricated by standard positive-resist electron beam lithography by patterning a 50- or 25-nm thick Au on a 1-nm Ti adhesive layer, which had first been evaporated onto an ultra-smooth fused silica substrate (1 × 2 cm 2 , surface finish 10/5, SVM). The diameters and gaps of the quadrumers were determined by top-view s.e.m. images, and heights were determined by 60° tilted-view s.e.m. images (divided by cos 60°). The standard deviations (error bars) were calculated based on 20 quadrumers. The fabricated quadrumers were arranged in a 7 × 7 array with 6 μm intercluster distances to avoid coupling effects. The substrate was treated with an oxygen plasma (660 W, Fischione) for 250 s for the removal of residual molecules before experimental use. SECARS experimental setup A sample-scanning nonlinear optical microscope was constructed for the single-particle SECARS measurements ( Supplementary Fig. 3 ). An ultrafast Ti:sapphire laser (Mira 900, Coherent Inc.) was used to generate the 800 nm pulses (repetition rate 76 MHz). After passing through a Faraday isolator (EOT Inc.), which allowed only one-way transmission of light, the laser beam was split into two paths. One path formed the pump beam at 800 nm with 5 nm FWHM by two band-pass filters (FB800-10, Thorlabs); the other path generated the Stokes beam at 830–1,050 nm by a nonlinear photonic crystal fibre (FemtoWhite800, Crystal Fiber A/S) for the Vis-NIR supercontinuum and then passed through a long-pass filter (BLP01-830R-25, Semrock). For each path, the polarization was controlled by a half-wave plate (10RP52-2, Newport) and a linear polarizer (LPVIS100, Thorlabs), and the intensity was attenuated by a neutral density filter (NDL-25C-4, Thorlabs). These two beams were then superimposed spatially using a dichroic mirror (DMSP805, Thorlabs). A motorized linear stage (ILS200CHA, Newport) was inserted into the Stokes path to overlap the pulses in time (pulse durations: pump ~200 fs; Stokes~500 fs). The collinear, coherent beams were then focused to ~1 μm diameter on an individual quadrumer using a × 50/0.8NA objective (HC PL FLUOTAR, Leica). Substrates were mounted on a three-axis piezoelectric stage (P-545.3R2 NanoXYZ, Physik Instrumente (PI) GmbH) to position the desired quadrumer precisely at the beam focus. The SECARS signal from the molecules was collected by a 60 × /0.7NA microscope objective with a variable coverslip correction collar (LUCPlanFL N, Olympus), then transmitted through a pair of short-pass filters (FF01-775/SP-25 and SP01-785RU-25, Semrock) to remove the excitation light. The light was focused onto the entrance slit of a spectrograph (SpectraPro 400i, PI/Acton) by an f =40 mm cemented achromatic doublet lens (AC254-040-A, Thorlabs), and detected by a Si CCD array (PIXIS 100, PI/Acton). The SECARS polarization was analysed by an additional polarizer (LPUV100, Thorlabs). A pair of CCD cameras (Guppy F-146, AVT and UI-2230-C-HQ,IDS) was used to obtain images of the back-scattered and transmitted light to assist in locating the specific quadrumer of interest on the substrate. Typically, SECARS experiments were performed with a total power of 40–100 μW for ensemble molecules or 600 μW for single molecules, corresponding to a power density of 4–10 kW cm −2 or 60 kW cm −2 (peak power density 0.13–0.325 GW cm −2 or 1.95 GW cm −2 ). Powers in both cases are smaller than those used in typical SERS experiments (>100 kW cm −2 ), but are capable of taking a full SECARS spectrum (−700 to −2,000 cm −1 ) within a short time (<1 s). Ensemble-molecule adsorption The substrates were soaked in a 10 mM p -MA (4-aminothiophenol, H 2 NC 6 H 4 SH, 97%, Aldrich) ethanolic solution, a 1 mM adenine (C 5 H 5 N 5 ,≥99%, Sigma) or benzocaine (C 9 H 11 NO 2 , Sigma) aqueous solutions overnight. A monolayer of p -MA molecules are believed to self-assemble onto the Au quadrumer surface and to bind to the substrate via the strong Au-S bond. Adenine and benzocaine molecules attach to the Au surface due to the Au-NH 2 bond. These substrates were then washed thoroughly to remove unattached molecules from the Au substrate before measurement. Linear optical measurements Dark-field scattering spectra were obtained by a custom-built microscope with 35° incidence from the substrate normal (Microscope: Axiovert 200 MAT, Zeiss; Objective: 50 × /0.55NA Epiplan-Neofluar, Zeiss; Spectrograph: SP2150, PI/Acton; CCD: PIXIS 400BR, PI/Acton). Simulation method Finite-difference-time-domain simulation commercial software (Lumerical FDTD Solutions 7.5.3) was used to obtain the near- and far-field properties of the quadrumer for normal incidence excitation. The top-view geometries were chosen to correspond as closely as possible to the experimentally obtained s.e.m. images of the quadrumer structures, and the heights used in the simulations corresponded to the Au thickness deposited during sample fabrication. A 1.3-nm thick dielectric layer on the side and top surfaces of each disk was used to model the p -MA monolayer. The Johnson and Christy dielectric function [42] was used for Au, ε 1 =2.10 for the infinite fused silica substrate, and ε 2 =9 for the p -MA molecules [23] . Charge density plots were obtained by calculating the difference of the normal component of the electric field above and below the Au surface (Gauss’s law). Single-molecule deposition A volume 25 ml of 200 nM p -MA ethanolic solution and 25 ml of 200 nM adenine aqueous solution were combined and mixed thoroughly. Then 10 μl of such mixture solution was drop-casted onto the SECARS substrate (1 × 2 cm 2 ), soaking the entire substrate surface and evaporating in ~2 s, such that on average an estimated number of ~0.75 p -MA and 0.75 adenine molecules fell into each probe region (~250 nm 2 area) of the substrate. This substrate was dried in air overnight to immobilize the probe molecules on the substrate surface, then dried under nitrogen flow before the SECARS measurements. How to cite this article: Zhang, Y. et al. Coherent anti-Stokes Raman scattering with single-molecule sensitivity using a plasmonic Fano resonance. Nat. Commun. 5:4424 doi: 10.1038/ncomms5424 (2014).